Evolutionary history predicts the stability of cooperation in microbial communities Cooperation fundamentally contributes to the success of life on earth, but its persistence in diverse communities remains a riddle, as selfish phenotypes rapidly evolve and may spread until disrupting cooperation. Here we investigate how evolutionary history affects the emergence and spread of defectors in multispecies communities. We set up bacterial communities of varying diversity and phylogenetic relatedness and measure investment into cooperation (proteolytic activity) and their vulnerability to invasion by defectors. We show that evolutionary relationships predict the stability of cooperation: phylogenetically diverse communities are rapidly invaded by spontaneous signal-blind mutants (ignoring signals regulating cooperation), while cooperation is stable in closely related ones. Maintenance of cooperation is controlled by antagonism against defectors: cooperators inhibit phylogenetically related defectors, but not distant ones. This kin-dependent inhibition links phylogenetic diversity and evolutionary dynamics and thus provides a robust mechanistic predictor for the persistence of cooperation in natural communities. Many unicellular organisms show complex social behaviours in which individuals actively communicate and cooperate [1] . Several bacteria secrete diffusible compounds that function as public goods benefiting all present organisms independently of their investment. Public goods include iron-scavenging siderophores [2] , extracellular enzymes [3] or secondary metabolites harming competitors and predators [4] . Such cooperative traits improve growth rate, competitiveness and virulence of pathogens. However, if the cooperative traits are costly, they may also be vulnerable to exploitation by cheats reaping benefits without sharing the costs [5] . Defectors have been reported to win over cooperators over a broad range of frequencies, calling for mechanisms explaining the persistence of cooperation [6] . Many bacteria use quorum sensing (QS) signalling to adjust the investment into public goods to the potential benefits [7] , [8] . Investment in QS-regulated traits typically increases with population density [8] , allowing to maximize benefits-to-costs ratio by investing in social behaviour in the presence of cooperating neighbours. This increased investment, however, is susceptible to cheating. In bacteria, defectors may emerge by evolution of signal blindness [9] , where an individual stops responding to QS signals [10] . Defectors’ fitness typically depends on the investment of cooperators into public goods [11] . Rare defectors may therefore show a high fitness [12] and invade if cooperators do not selectively enforce cooperation by harming defectors [13] . The establishment and stability of cooperation have been extensively studied using single pairs of cooperators and defectors, predicting defector’s fitness as a function of cooperators investment in public goods and spiteful behaviours [14] . Most studies use the Hamiltonian kin selection framework [15] predicting that altruism becomes evolutionary stable as relatedness augments. In a multispecies system, this concept can be extended to evolutionary history: because of their common ancestry, different species may share compatible kin recognition mechanisms and perceive each other as partner, although differing at the level of the cooperative locus [16] , [17] . Bacteria live in complex communities forming networks of antagonistic or facilitative interactions [18] , [19] , with very little being known on the dynamics of cooperative behaviours in multispecies microbial communities. Diversity does not impede cooperation per se [20] , but makes it difficult to predict using the Hamiltonian framework. In multispecies communities, cross-talk between unrelated species may result in cooperative behaviour [17] . Further, antagonistic interactions, as caused by the production of bacteriocins or antibiotics, may harm a broad range of competitors [21] , independent of their cooperativeness or shared evolutionary history with the emitter strain [22] . We investigated how biodiversity affects the stability of cooperation. We set up mixed communities ranging from one to eight Pseudomonas spp. genotypes, a model taxon in ecological and evolutionary research [3] , [23] . The communities varied in two diversity metrics, the richness (number of genotypes) and evolutionary history (mean pairwise phylogenetic distance), two widely used indices with contrasting effects on community performance [24] . We grow the bacteria in quorum sensing medium (QSM) [3] , a minimal medium with albumin as the sole carbon source. Albumin first has to be degraded by extracellular proteases, which function as a QS-regulated public good in Pseudomonas [25] . Fluorescent pseudomonads produce extracellular proteases under the control of the gac–rsm QS system and may respond to their own as well as other species’ QS signals [17] , [25] . We monitor the apparition of spontaneous protease-deficient defectors in communities of varying phylogenetic history and richness. We expect that if high genetic relatedness between strains promotes their ability to cooperate, community phylogenetic history will predict the fate of cooperation. On the other hand, if non-additive diversity effects drive the fitness of defectors [24] , we expect that community richness would be the best predictor of the stability of cooperation. We further set up a second experiment with a focal-defined defector and followed its fitness as a function of its original frequency, community richness and mean phylogenetic distance between the defector and surrounding cooperators. We then analyse if biodiversity effects on defector success can be attributed to the investment into public goods and defector inhibition by the cooperating genotypes. We observe that the stability of cooperation is directly proportional to the mean phylogenetic relatedness between the present genotypes. Communities containing phylogenetically close species keep cooperating, whereas communities containing phylogenetically distant species get rapidly invaded by defectors emerging by spontaneous mutation. We show that this pattern is due to antagonistic interactions, as cooperators can inhibit defectors from closely related genotypes but not from unrelated ones. Spread of evolved defectors In this first experiment, multispecies communities of cooperators are growing on albumin as the sole carbon source. Bacteria must produce proteases to break down and assimilate the nutrients. In pseudomonads, protease-deficient mutants rapidly emerge by mutation of the gacS/gacA QS cascade [26] . In our experiment, protease-deficient phenotypes rapidly evolve out of initially cooperating communities. Their spread is further closely correlated to the mean pairwise phylogenetic distance (generalized linear model (GLM), F 1,46 =112.1, P <0.001; Fig. 1 ), but not to the richness (GLM, F 1,46 =0.8, P =0.36 when fitted sequentially after mean pairwise phylogenetic distance) of the community: although communities of phylogenetically related bacteria remain virtually free of defectors, phylogenetically diverse communities rapidly accumulate protease-deficient defectors. None of these defector isolates could grow on QSM alone, even with addition of signals from the cooperators, suggesting that these were signal-blind defectors relying on the public goods (proteases) secreted by the cooperators. The phenotype of the isolated defectors is typical for mutations in the gacS/gacA QS cascade [27] , a rapidly mutating system whose deactivation results in signal blindness and accounts for virtually all protease-deficient mutants in Pseudomonas spp. [9] , [28] . 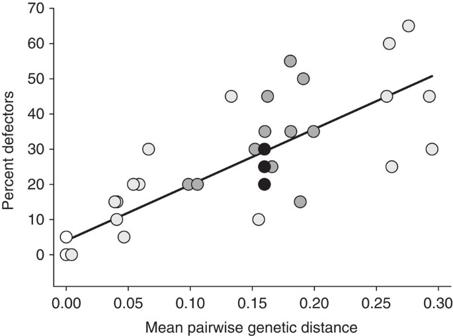Figure 1: Effect of the mean pairwise genetic distance ofPseudomonasspp. communities on the emergence and spread of signal-blind defectors. Communities (100% cooperators at the beginning of the experiment) were grown on QSM medium for 48 h. Signal-blind defectors were discriminated by their lack of proteolytic and tryptophan dioxygenase activity and expressed as per cent of the community after 48 h (GLM,R2=0.72,P<0.001). Symbol shading shows the richness of the different communities: white, monocultures; light grey, two genotypes; dark grey, four genotypes; and black, eight genotypes. Figure 1: Effect of the mean pairwise genetic distance of Pseudomonas spp. communities on the emergence and spread of signal-blind defectors. Communities (100% cooperators at the beginning of the experiment) were grown on QSM medium for 48 h. Signal-blind defectors were discriminated by their lack of proteolytic and tryptophan dioxygenase activity and expressed as per cent of the community after 48 h (GLM, R 2 =0.72, P <0.001). Symbol shading shows the richness of the different communities: white, monocultures; light grey, two genotypes; dark grey, four genotypes; and black, eight genotypes. Full size image As defector fitness may be related to the cooperators’ investment into public goods [11] , we further test if the defector load is correlated with the proteolytic activity of the community. Under the tested conditions, proteolytic activity is unaffected by the genetic distance between the genotypes present (GLM, R 2 =0.01, P =0.90), suggesting that phylogenetically distant genotypes engage into cooperative behaviours. Proteolytic activity only partially predicts defector load (GLM, R 2 =0.10, P =0.04), suggesting that other interactions such as antagonistic ones may drive the fitness of emerging defectors. Phylogenetic constraints on defector inhibition To uncover antagonistic interactions, we investigate if cooperators selectively harm defectors and if harming is affected by phylogenetic distance. In bacteria, inhibition of competitors often relies on diffusible toxins [29] , prompting us to test if cooperators secrete metabolites harming defectors. We use an isogenic signal-blind mutant of one of the used genotypes ( Pseudomonas fluorescens CHA0Δ gacS [30] ) as model defector of defined genetic background. This mutant is typical for spontaneous mutations deactivating secondary metabolism in pseudomonads [28] and lacks extracellular proteases required for growing on albumin [3] , [30] . It grows better than the wild type when cooperation is not required [4] , but preliminary experiments showed that it is incapable of growing on QSM medium alone. In order to investigate its growth inhibition by the cooperators, we grow this mutant under non-limiting nutrient conditions (Lysogeny Broth (LB)) supplemented with small amounts of supernatant from communities grown in QSM. Supernatants inhibit the growth of the signal-blind mutant and the inhibition is negatively correlated with the mean phylogenetic distance between the community and the defector (GLM, R 2 =0.44, P <0.001; Fig. 2 ), but not to community richness (GLM, R 2 =0.08, P =0.4). To exclude effects due to the genetic background, we also assess the response of the wild-type CHA0, with no significant effect of phylogenetic distance on its growth (GLM, R 2 =0.01, P =0.9). These results suggest that cooperators produce diffusible toxins specifically suppressing phylogenetically close defectors. 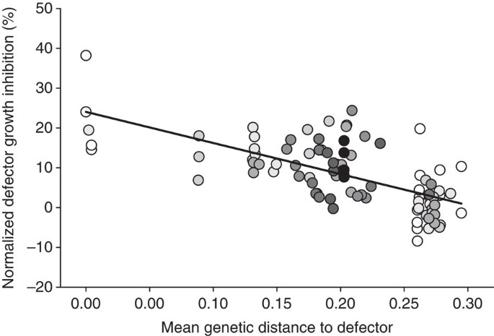Figure 2: Relationship between phylogenetic distance and defector inhibition. Effect of mean genetic distance between the defector and the community of cooperating bacteria on the growth inhibition of the model defectorPseudomonas fluorescensCHA0ΔgacSby cell-free supernatant of a 48-h-old cooperator cultures varying in mean genetic distance to the defector (GLM,R2=0.44,P<0.001). Inhibition was expressed as the growth reduction compared with control, normalized by the growth reduction of the wild-type background genotype CHA0. Note that to improve the robustness of the prediction, 96 communities were tested instead of the 48 used in the competition experiment. Symbol shading shows the richness of the different communities, ranging from white (monocultures) to black (eight genotypes). Figure 2: Relationship between phylogenetic distance and defector inhibition. Effect of mean genetic distance between the defector and the community of cooperating bacteria on the growth inhibition of the model defector Pseudomonas fluorescens CHA0Δ gacS by cell-free supernatant of a 48-h-old cooperator cultures varying in mean genetic distance to the defector (GLM, R 2 =0.44, P <0.001). Inhibition was expressed as the growth reduction compared with control, normalized by the growth reduction of the wild-type background genotype CHA0. Note that to improve the robustness of the prediction, 96 communities were tested instead of the 48 used in the competition experiment. Symbol shading shows the richness of the different communities, ranging from white (monocultures) to black (eight genotypes). Full size image Frequency-dependent defector fitness To validate if defector inhibition rather than investment into public goods may explain the low defector load of phylogenetically related communities, we model and test experimentally frequency-dependent fitness of defectors under various cooperation and harming scenarios. We simulate defector payoff at different initial frequencies with a modified snowdrift model [31] . This game theory model considers payoff of defection as a function of the investment of the whole community into public goods. We complete this model by adding a defector inhibition function based on fully diffusible toxins. Assuming that QS regulates the production of both public goods and toxins [25] , the per capita and population-level investment in these two traits will increase as a linear [32] and quadratic function of cooperator frequency, respectively. The model predicts that payoff (benefits minus costs) of defection will be negatively frequency dependent in the absence of specific inhibition of the defectors ( Fig. 3a ), and reflects well previous studies on the negative frequency-dependent fitness of defectors [12] . As this inhibition increases, payoff becomes hump-shaped, resulting in the defector to go extinct except at intermediate frequency. As the toxin function peaks at low defector frequency, low toxicity of the cooperators towards the defectors is sufficient to annihilate the advantage of rare defectors, stabilizing cooperation by preventing emerging defectors from invading ( Fig. 3a ). 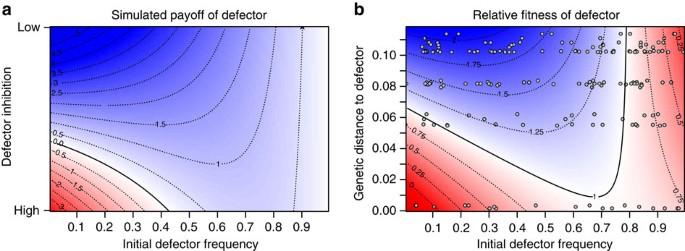Figure 3: Simulation and empirical data on defector fitness under increasing defector inhibition. (a) Simulation of defector payoff as a function of defector initial frequency and presence of compounds specifically inhibiting defectors. A positive relative payoff (blue region) indicates higher fitness of the defector, whereas a negative one indicates higher fitness of the cooperator (red region). (b) Empirical data showing the fitness of the model defectorPseudomonas fluorescensCHA0ΔgacSas a function of its initial frequency and its mean genetic distance to the community of cooperating bacteria. A fitness value >1 (blue region) indicates faster growth of the defector, whereas a value between 0 and 1 (red region) indicates faster growth of the cooperator. The isoclines correspond to the polynomial surface regression reported inTable 1(R2=0.56,P<0.0001). Grey circles represent the individual communities. Figure 3: Simulation and empirical data on defector fitness under increasing defector inhibition. ( a ) Simulation of defector payoff as a function of defector initial frequency and presence of compounds specifically inhibiting defectors. A positive relative payoff (blue region) indicates higher fitness of the defector, whereas a negative one indicates higher fitness of the cooperator (red region). ( b ) Empirical data showing the fitness of the model defector Pseudomonas fluorescens CHA0Δ gacS as a function of its initial frequency and its mean genetic distance to the community of cooperating bacteria. A fitness value >1 (blue region) indicates faster growth of the defector, whereas a value between 0 and 1 (red region) indicates faster growth of the cooperator. The isoclines correspond to the polynomial surface regression reported in Table 1 ( R 2 =0.56, P <0.0001). Grey circles represent the individual communities. Full size image We validate the model by growing the signal-blind CHA0Δ gacS at various initial frequencies in QSM with the bacterial communities described above. Defector fitness matches the predictions from the model: in the presence of phylogenetically distant (and thus inefficiently inhibiting defectors) cooperator communities defector fitness is negatively frequency-dependent ( Fig. 3b ). This corresponds well to predictions of defector fitness without antagonistic interactions [12] . Fitness is particularly high at low frequency, where small numbers of defectors can exploit large amounts of public goods, so that evolved defectors can rapidly invade. In contrast, the fitness of the mutant facing phylogenetically close (and efficiently inhibiting defectors) cooperators is hump-shaped and peaks at intermediate frequency with rare mutants having very low fitness and being unable to invade ( Fig. 3b ). Mutant fitness can be well predicted as a function of its initial frequency and mean phylogenetic distance to the remaining community ( Table 1 ). Defector inhibition is the best predictor of mutant fitness (initial frequency × defector inhibition interaction; Table 1 ), surpassing the effect of public good production (proteolytic activity). Table 1 Effects of phenotypic traits and genetic structure on the fitness of the defector. Full size table Biodiversity is an important driver of ecological processes. In this study, we show that evolutionary history also predicts the stability of cooperation in multispecies communities ( Fig. 4 ). Interestingly, investment in public goods (proteases) was independent of the phylogenetic distance within the community. The gac/rsm QS pathway is highly conserved among Pseudomonas spp. [25] , and phylogenetically distant species engage in cooperation due to an overlap in QS signals [17] . Using ’leaky’ communication systems open to cross-talk may be a powerful way of optimizing cooperation as resource differentiation between competitors positively correlates with phylogenetic distance [24] . In an ideal scenario, distant species cooperate making a common resource available. Each species then uses different resource fractions thereby reducing competition. In this scenario, a phylogenetically closely related defector is more threatening than an unrelated cooperator, as it is not contributing to opening up resources but resource consumption may highly overlap with the cooperator. In agreement with this conflict, defector inhibition decreased with increasing phylogenetic distance. Cooperators rapidly evolve mechanisms that prevent defection [33] , and in our experiment the ability of cooperators to constrain the emergence of defectors is closely linked to their genetic relatedness. Owing to the high rate of QS disrupting mutations [9] , [27] and the fact that the emerging mutants are imbedded in populations of the cooperating parental strain, the necessity of the parental strain to control the spread of defecting clone mates likely exceeds that of controlling invasion by unrelated defectors. Invasion by unrelated defectors occurs from outside the population, whereas signal-blind defector mutants emerge by cell division inside the population of the cooperating ancestor. Based on our results, we propose that inhibition of closely related defectors was due to a combination of policing, in which cooperators invest into harming of defectors [34] , and disruption of QS via pleiotropic effect reducing resistance to various biotic and abiotic stressors [4] , [35] . The increased sensitivity of defectors to genetically related cooperators points to a suppression of close kin refusing to cooperate. This resembles policing in social Hymenoptera suppressing reproductive workers that reinforces cooperation once established [36] ; however, in social Hymenoptera policing increases with genetic distance [37] whereas in P. fluorescens it is most pronounced against closely related defectors. As a result, mixtures of closely related genotypes will stably cooperate because the emerging defector suffers from toxins of all the clonal and close kin cells of the parental strain. Mixtures of more distant genotypes will still cooperate, but will not be able to control the emergence of defectors. 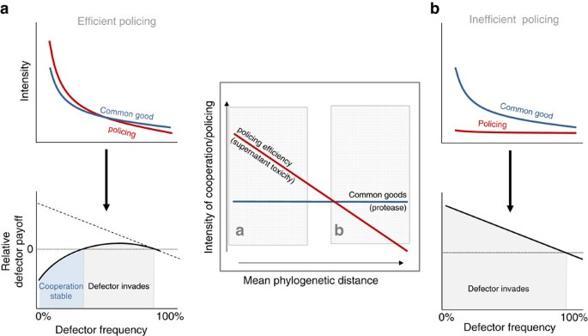Figure 4: Conceptual representation of the mechanisms linking evolutionary history and the stability of cooperation. We observe that defector inhibition is the main predictor of defector spread. As phylogenetic distance between competing species increase, the investment into cooperation remains stable, but the efficiency of defector inhibition decreases. Based on the mathematical prediction and the experimental data, this reduced inhibition favours the spread of defectors: in closely related communities (a), cooperators not only produce public goods but also toxins efficiently inhibiting defectors. Rare defectors (for example, emerging by mutation) face high toxicity cancelling the advantage of defection and cannot invade communities of cooperators. In contrast, in loosely related communities (b), rare defector profit from the high investment into public goods by the cooperators. Defector fitness is negatively frequency dependent, and rare defectors may invade. Functions for both public goods and defector inhibition are quadratic, reflecting thatper capitainvestment by cooperators is density-dependent (quorum-sensing-regulated). Figure 4: Conceptual representation of the mechanisms linking evolutionary history and the stability of cooperation. We observe that defector inhibition is the main predictor of defector spread. As phylogenetic distance between competing species increase, the investment into cooperation remains stable, but the efficiency of defector inhibition decreases. Based on the mathematical prediction and the experimental data, this reduced inhibition favours the spread of defectors: in closely related communities ( a ), cooperators not only produce public goods but also toxins efficiently inhibiting defectors. Rare defectors (for example, emerging by mutation) face high toxicity cancelling the advantage of defection and cannot invade communities of cooperators. In contrast, in loosely related communities ( b ), rare defector profit from the high investment into public goods by the cooperators. Defector fitness is negatively frequency dependent, and rare defectors may invade. Functions for both public goods and defector inhibition are quadratic, reflecting that per capita investment by cooperators is density-dependent (quorum-sensing-regulated). Full size image Overall, the results suggest that uncoupling of phylogeny and cooperation helps in explaining one of the major riddles in evolutionary biology: the stability of cooperation. Cooperation is facilitated by kin selection as genetically related organisms share genes. However, related organisms also occupy similar niches and use similar resources, which increases competition [38] . Evolutionary history has been shown to drive the productivity of plant and microbial communities [24] , [39] , and we show that it may also affect the evolution of new phenotypes. Suppression of genetically related defectors was the major determinant of the stability of cooperation in multispecies microbial communities. Increasing phylogenetic distance between the species of a community did not directly decrease investment into cooperation, but rather the ability of the cooperators to control the spread of defectors. The number of genotypes present did not affect the relationship between phylogenetic distance and defector fitness, suggesting that this study may serve to predict the fate of cooperation in more complex communities. Therefore, the present study links phylogenetic structure to evolutionary dynamics of bacterial communities, providing a mechanistic understanding of the stability of cooperative behaviours in complex multispecies communities. Organisms and set-up of bacterial communities We used the eight well-characterized Pseudomonas spp. genotypes CHA0, PF5, Q2-87, 1M1-96, Q8R1-96, MVP1-4, F113 and Phl1C2 (ref. 40 ). Although classified as P. fluorescens , recent comparative genomics studies indicate that they belong to at least three species [41] . Forty-eight communities were assembled from the eight genotypes, covering a richness of one (each of the eight genotypes in monoculture with two replicates each), two (16 combinations), four (12 combinations) and eight genotypes (4 replicates), according to a previously published design [19] . Also, these communities span a gradient in phylogenetic relatedness (see below). All genotypes were assessed for production of exoprotease as model public good. Bacteria were grown overnight in LB, pelleted by centrifugation and washed three times in 0.85% NaCl to remove nutrients. Bacteria were mixed to set-up the desired communities (total of 2 × 10 7 bacteria per community). Emergence of evolved defectors Bacteria were grown in QSM [3] , a minimal medium containing 1% bovine serum albumin as the sole carbon source, at 25 °C with agitation for 48 h. This time lapse corresponds to about 25 generations and is known to allow the evolution and spread of new phenotypes [28] . Bacteria were serial-diluted and enumerated on milk agar plates (tryptic soy broth 3 g l −1 , agar 15 g l −1 and skim milk 150 ml l −1 ). In Pseudomonads, protease-negative phenotypes emerge as a consequence of deactivation of the gac–rsm QS cascade [9] , [28] . To confirm that ’defectors’ were not simply protease-deficient mutants, we looked for colonies lacking, in addition to proteolytic activity, tryptophane dioxygenase activity, another trait regulated by the gac–rsm pathway [27] . Three days old colonies were screened for proteolytic (transparent halo around the colony) and tryptophan dioxygenase activity (brown colouration when overlaid with tryptophane [42] ). We counted colonies lacking exoproteases and tryptophan dioxygenase as signal-blind defectors [27] . In order to further test if these mutants are signal blind, we randomly picked 20 protease-deficient isolates and attempted to grow them in QSM medium with or without an organic extract from wild-type cultures (containing QS signals) as described elsewhere [17] . Frequency-dependent fitness of signal-blind defectors We used the isogenic signal-blind mutant CHA0Δ gacS , chromosomally tagged with green fluorescent protein [43] . This mutant lacks QS and lacks extracellular proteases required for growth on proteins [30] . Signal blindness is predicted to be the most advantageous defection strategy [10] , and is the most common mechanism of defection from QS-regulated traits in pseudomonads [9] . Forty-eight microbial communities were assembled as described above and mixed with the defector CHA0Δ gacS -green fluorescent protein at frequencies of 10%, 33%, 66% and 90% defector. The OD 600 of the whole community including defector was adjusted to 0.05 in 200 μl QSM. A total of 192 communities were established (48 communities × 4 defector frequencies) and grown with agitation at 25 °C for 36 h (early stationary growth phase). At the beginning and at the end of the experiment, bacteria were enumerated using a C6 Flow Cytometer (Accuri). Total bacteria were gated on the base of their forward scatter (FSC) side scatter (SSC) signal, defectors on the base of the FL1-A signal (green fluorescence). The relative fitness ω of the defector was calculated from the ratio of Malthusian growth parameters: ω= ln ( X final / X initial )/ln( Y final / Y initial ), where X and Y are the concentrations (number of bacteria ml −1 ) of the defector and the remaining community, respectively [3] . Relative fitness >1 indicates superior growth of the defector. Phylogenetic relationships Phylogenetic distance was estimated on the base of the phlD nucleotide sequence, a functional gene coding for a polyketide synthase present in all tested genotypes. This gene provides a robust estimator of phylogenetic distance among the studied bacteria [44] and correlates well with metabolic differentiation [24] . Genetic distance between the genotypes was calculated with the Kimura algorithm using the dna.dist() function (package ’ape’) in R. Mean genetic distance between the defector and the remaining community was defined as MGD x = , where ‘Dist’ is the genotypic distance between the defector x and the cooperator y , and P the relative abundance of y in the community. The mean pairwise genetic distance between genotypes present in a community was defined as MGD tot = . MGD tot is equivalent to ‘genotypic dissimilarity’ in previous studies [24] . See Fig. 5 for a detailed view of the interrelationships between diversity indices and a neighbor-joining phylogenetic tree of the used genotypes. 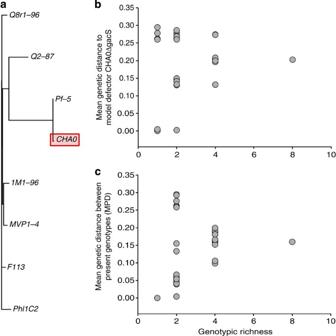Figure 5: Phylogenetic relationships between the differentPseudomonasspp. genotypes and communities used in this study. (a)phlD-based neighbour-joining tree of the eight used genotypes. (b) Relationship between community richness (number of genotypes) and the mean pairwise distance between the present genotypes and the model defectorPseudomonas fluorescensCHA0ΔgacS. (c) Relationship between the community richness and mean pairwise phylogenetic distance between the genotypes. Figure 5: Phylogenetic relationships between the different Pseudomonas spp. genotypes and communities used in this study. ( a ) phlD -based neighbour-joining tree of the eight used genotypes. ( b ) Relationship between community richness (number of genotypes) and the mean pairwise distance between the present genotypes and the model defector Pseudomonas fluorescens CHA0Δ gacS . ( c ) Relationship between the community richness and mean pairwise phylogenetic distance between the genotypes. Full size image Public good and toxin production We tested the ability of the studied genotypes grown alone or in mixture to inhibit the growth of the signal-blind mutant CHA0Δ gacS [30] by establishing a total of 96 communities ranging from one to eight genotypes [24] . Each community was grown in QSM as described above, the bacteria were pelleted by centrifugation (15,000 g , 5 min) and the supernatant was sterile filtered. Growth inhibition was assessed by mixing a liquid culture of CHA0Δ gacS in 135 μl 1/10 LB (OD 600 =0.05) supplemented with 15 μl of sterile filtered supernatant. Controls received sterile albumin-free QSM. Toxicity was rated as the relative growth inhibition of the defector at 25 °C after 24 h. To ensure that the observed growth inhibition patterns were caused by signal blindness and not by the sensitivity of the parent genotype, we repeated the measurements with P. fluorescens CHA0 as test organism. Public goods (extracellular proteases) were defined as the proteolytic activity in sterile filtered supernatant of each community, as measured with an azocasein assay [45] . Modelling of defector fitness To test if the observed patterns of public goods and defector-inhibiting toxins may explain defector fitness, we added a defector inhibition function to an existing snowdrift model [31] . We modelled the relative payoff P of an individual x in a mixed community as P ( x , y ) = B ( x + y ) – C b ( x ) – C t ( x ) – E × T ( y , x ) , with B the benefit function of the total investment in public goods, C b and C t the cost function for public goods and toxins, and T the toxicity function for toxins produced by y , showing an efficiency E against x . Considering that the toxins only affect the defector and that defectors neither produce public goods nor toxins ( C b ( x ) = C t ( x ) =0), the payoff of the defector x can be simplified to P ( x ) = B ( x + y ) – E × T ( y , x ) and the payoff of the cooperator y to P ( y ) = B ( x + y ) – C b ( y ) – C t ( y ) (ref. 31 ). In order to reflect that QS-regulated traits are density-dependent [13] , [14] , we assume the per capita investment of the cooperator y to linearly increase with frequency, so that the B ( y ) , C b ( y ) and C t ( y ) functions are quadratic functions of cooperator frequency. If E × T ( y , x ) > C b ( x ) + C t ( x ) , the advantages of defecting are counterbalanced by inhibition, resulting in higher relative payoff of cooperators ( P ( x ) − P ( y ) <0). At low defector frequency, cooperators will invest more in anti-defector toxins, which may harm rare defectors and cancel the benefits of defection. We explored different parameter combinations consistently showing a transition from a negative frequency-dependent to a hump-shaped defector fitness curve as E increases, indicating that rare defector mutants may be unable to invade communities of cooperating bacteria efficiently harming them ( Fig. 3 ). Statistical analyses We analysed the effects of initial defector frequency (continuous), genotypic richness of the community of cooperators (categorical) and genetic distance between defector and the remaining community of cooperators (continuous) on defector fitness with a polynomial GLM. For more precision, we used the measured initial defector frequency in each single community and not the set-up one, justifying its use as continuous factor (see Fig. 2b ). Using the same approach, the effect of the production of proteases (public good) and specific defector growth reduction (inhibition efficiency) on defector fitness was assessed. To account for the imperfect orthogonality between the diversity indices ( Fig. 5 ), we fitted richness and mean phylogenetic distance in a sequential GLM. Sequential GLM is a common statistical approach to test several inter-related biodiversity measures in one model [46] . The effects of genotypic richness and genetic distance between the defector and the community of cooperators were further tested against bacterial composition in order to avoid pseudo-replication [24] , [46] . How to cite this article: Jousset, A. et al. Evolutionary history predicts the stability of cooperation in microbial communities. Nat. Commun. 4:2573 doi: 10.1038/ncomms3573 (2013).